Multi-octave supercontinuum generation from mid-infrared filamentation in a bulk crystal In supercontinuum generation, various propagation effects combine to produce a dramatic spectral broadening of intense ultrashort optical pulses. With a host of applications, supercontinuum sources are often required to possess a range of properties such as spectral coverage from the ultraviolet across the visible and into the infrared, shot-to-shot repeatability, high spectral energy density and an absence of complicated pulse splitting. Here we present an all-in-one solution, the first supercontinuum in a bulk homogeneous material extending from 450 nm into the mid-infrared. The spectrum spans 3.3 octaves and carries high spectral energy density (2 pJ nm −1 –10 nJ nm −1 ), and the generation process has high shot-to-shot reproducibility and preserves the carrier-to-envelope phase. Our method, based on filamentation of femtosecond mid-infrared pulses in the anomalous dispersion regime, allows for compact new supercontinuum sources. Coherent ultra-broadband light sources are in demand for a variety of applications. Modern imaging exploits broadband light to map biological materials with high spatial resolution. Multi-photon spectroscopy and microscopy demand focussable and coherent light at a variety of wavelengths enabling, for example, chemical-specific imaging of biological samples. Modern nonlinear spectroscopy [1] benefits from time-resolved multi-colour pump-probe capabilities for tracking the motion of valence electrons and nuclei on their natural femtosecond timescale. Spectroscopy in the molecular fingerprint regions of the mid-infrared [2] has promising applications such as breath analysis for medical diagnosis. Frequency combs [3] , [4] in the visible to mid-infrared enable ultrahigh resolution spectroscopy used, for example, to study the composition of extrasolar planets. Finally, coherent supercontinua are a step towards arbitrary multi-colour waveform synthesis, which offers simultaneous probing and control [5] of electronic, vibrational and rotational motion, or synthesizing single electric-field waveforms at arbitrary carrier wavelengths [6] . These applications place widely varying demands on the characteristics of a supercontinuum source. Novel optical fibres yield supercontinua spanning the ultraviolet into the mid-infrared [7] , [8] , [9] . Besides the intrinsic peak power limitations and alignment sensitivity, the most extreme bandwidths observed in fibres have been achieved at the expense of pulse-to-pulse repeatability, which often manifests in complicated temporal pulse splitting and fine spectral modulation [8] , [10] . A requirement for shot-to-shot repeatability and a smooth spectrum therefore limits the allowable propagation length, restricting the bandwidth significantly [8] . Alternatively, spectral broadening of visible and near-infrared drivers in bulk materials has thus far not achieved bandwidths comparable to those from fibres, and long wavelength extensions of the spectrum are inefficient and require extreme conditions [11] , [12] , [13] . This suggests the necessity of increasing the pump wavelength to extend the long wavelength edge of the supercontinuum, but raises the question of whether a corresponding increase in the short wavelength edge will occur. Here we present a supercontinuum produced by filamentation of femtosecond mid-infrared pulses in bulk yttrium aluminium garnet (YAG) crystal. The spectrum spans 450–4,500 nm, the broadest ever produced by filamentation in bulk. We verify carrier-envelope phase stability and shot-to-shot repeatability. Simulations indicate an absence of complex pulse splitting and self-compression of the pump pulse by a factor of 10. Angularly resolved spectrum The pump pulses were produced with an optical parametric chirped pulse amplifier, which delivered carrier-envelope phase stable, 85 fs pulses at 3,100 nm centre wavelength and with a repetition rate of 160 kHz (ref. 14 ). The set-up for generating and measuring the supercontinuum is shown in Fig. 1 . Pulses of 6.9 μJ energy were collimated to 4 mm diameter and were focussed by a 75-mm focal length CaF 2 lens to a 1/ e 2 diameter of 50 μm. The peak power was 76 MW, which is approximately three times above the critical power for YAG. The 2-mm-thick YAG plate was placed into the focal region, producing a clearly visible filament. We observed no irregular or interference patterns typically indicative of multifilamentation. At a distance of 54 mm after the exit plane of the YAG plate, we acquired an angularly resolved { θ , λ } spectrum that provided our connection to the theory and numerical simulations. Three optical fibres, each aligned parallel to the optical axis and displaced horizontally, delivered light to three spectrometers: a silicon charged-coupled device (CCD) spectrometer (Ocean Optics HR4000), an InGaAs CCD spectrometer (Ocean Optics NIR256), and a Fourier transform infrared spectrometer (Oriel MIR8025) with HgCdTe detector. The three fibre tips, moving as a single unit, were scanned horizontally in steps of 0.5 mm. At each step, data was acquired for 4 ms for the silicon CCD, 25 ms for the InGaAs CCD, and ~50 ms for the HgCdTe Fourier transform infrared spectrometer. We applied spectral intensity calibrations, taken with a black-body source, of the combined response of each fibre-spectrometer pair. A scaling factor was then applied to the data from each spectrometer to achieve consistency in their regions of overlap (925 and 2,500 nm) and with the measured pulse energy. The result is shown in Fig. 2a , along with a corresponding numerical simulation in Fig. 2b that we discuss below. 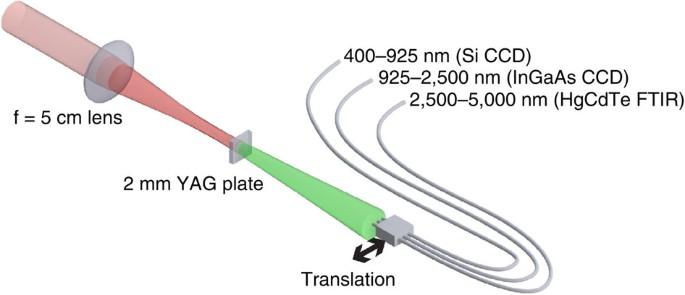Figure 1: Set-up for supercontinuum generation and measurement of its angularly resolved spectrum. Schematic of the generation and measurement set-up; the mid-infrared beam (red) is focussed by a 50-mm focal length CaF2lens. The supercontinuum (green) is generated in a 2-mm thick YAG plate and the {θ,λ} distribution is recorded by horizontally scanning three closely spaced fibres across the emerging beam. Figure 1: Set-up for supercontinuum generation and measurement of its angularly resolved spectrum. Schematic of the generation and measurement set-up; the mid-infrared beam (red) is focussed by a 50-mm focal length CaF 2 lens. The supercontinuum (green) is generated in a 2-mm thick YAG plate and the { θ , λ } distribution is recorded by horizontally scanning three closely spaced fibres across the emerging beam. 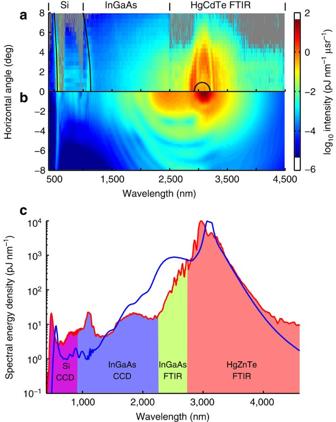Figure 2: Measured and simulated angularly resolved and angularly integrated spectra. (a) Measurement and (b) simulation of the far field {θ,λ} representation in absolute units; the grey area in (a) indicates the noise level, and the detector ranges are shown above the figure. Analytical results of a simple phase-matching picture are superimposed with black lines in (a). (c) Supercontinuum generated by 3,100 nm, 2.6 μJ pulses in YAG (red). The ranges of each spectrometer/detector are indicated and superimposed is the angle-integrated spectrum from our simulation (blue). Two different detectors (InGaAs and HgCdZnTe) were used to cover the long wavelength region. FTIR, Fourier Transform Infrared Spectrometer. Full size image Figure 2: Measured and simulated angularly resolved and angularly integrated spectra. ( a ) Measurement and ( b ) simulation of the far field { θ , λ } representation in absolute units; the grey area in ( a ) indicates the noise level, and the detector ranges are shown above the figure. Analytical results of a simple phase-matching picture are superimposed with black lines in ( a ). ( c ) Supercontinuum generated by 3,100 nm, 2.6 μJ pulses in YAG (red). The ranges of each spectrometer/detector are indicated and superimposed is the angle-integrated spectrum from our simulation (blue). Two different detectors (InGaAs and HgCdZnTe) were used to cover the long wavelength region. FTIR, Fourier Transform Infrared Spectrometer. Full size image Figure 2a shows that the long wavelength edge decays smoothly, reaching the noise level at 4,500 nm, while the short wavelengths extend to 450 nm. The highest spectral energy density is found around the mid-infrared pump wavelength with a maximum angularly-integrated spectral density of 10 nJ nm −1 . The smallest energy content is observed in the 750–1,000 nm range at a few picojoule per nanometer; these energies are still sufficient for most absorption spectroscopy experiments. We observe a structure at 610 nm in the { θ , λ } representation, whose energy content is roughly one order of magnitude higher than at the minimum at 850 nm with a feature clearly distinguished at 1,100 nm. Fig. 2c shows an alternative measurement by imaging the supercontinuum into each spectrometer fibre to improve the signal-to-noise ratio. This measurement featured a lower pulse energy but a tighter focus, leading to a slightly different spectrum extending down to 450 nm. For this measurement, two different detectors were used (InGaAs and HgCdZnTe) instead of the HgCdTe detector to cover the long wavelength region, as indicated by the shaded regions in Fig. 2c . We note that due to anisotropy of the third-order tensor in YAG, one would in general expect a rotation of the polarization during the supercontinuum generation. In our investigations of this effect, we found that the induced ellipticity is below 0.1 across the entire spectrum, with a weak dependence on the crystal orientation. The major axis remains aligned with the pump. The apparent weakness of anisotropic effects for our parameters justifies a scalar theoretical treatment and means that the usefulness of the source is not impacted by polarization scrambling. Shot-to-shot reproducibility A practical issue for applications of a supercontinuum, particularly considering the potential for few-cycle pulse generation, is the shot-to-shot reproducibility of the waveform. The process must therefore be deterministic and not excessively sensitive to the inevitable shot-to-shot fluctuations of the drive laser. These properties have been demonstrated in bulk supercontinuum generation with 800 nm pumping [15] , [16] , [17] , and we now show that they also hold for our mid-infrared pumping conditions using an f –2 f interferometer, shown in Fig. 3 . We recorded the spectral interference pattern formed by the supercontinuum and its second harmonic (further details in Methods). The phase of the fringes is sensitive to the carrier-envelope phase of the supercontinuum pulses, as well as their intensity fluctuations [15] . Figure 4 shows a 15-s subset of a dataset recorded over a 10-min interval. 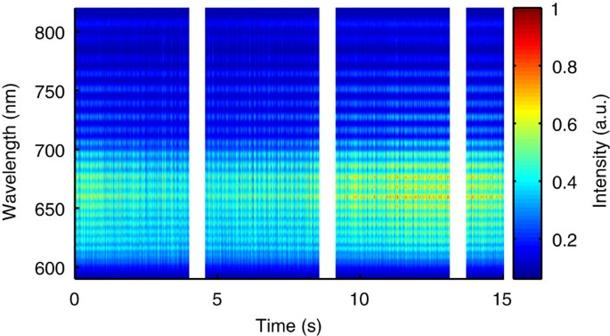Figure 4:f–2finterference fringes. Spectral interference fringes produced byf–2finterference between the long and short wavelength edges of the spectrometer over time. Over the full 10 min, the fringe phase has a standard deviation of 259 mrad (ref. 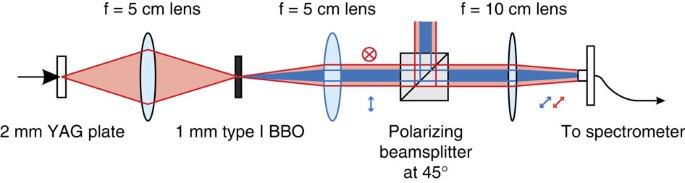14 ). Figure 3:f–2finterferometer for supercontinuum generation. Schematic of thef–2finterferometer for monitoring the stability of the supercontinuum. Red and blue beams represent the fundamental and the second harmonic, and the correspondingly coloured arrows represent the polarization state. The fundamental and its orthogonally polarized second harmonic, produced in a beta-barium borate crystal, are projected onto the same polarization state by a beamsplitter cube. Figure 3: f–2f interferometer for supercontinuum generation. Schematic of the f–2f interferometer for monitoring the stability of the supercontinuum. Red and blue beams represent the fundamental and the second harmonic, and the correspondingly coloured arrows represent the polarization state. The fundamental and its orthogonally polarized second harmonic, produced in a beta-barium borate crystal, are projected onto the same polarization state by a beamsplitter cube. Full size image Figure 4: f–2f interference fringes. Spectral interference fringes produced by f–2f interference between the long and short wavelength edges of the spectrometer over time. Full size image To connect the physics to the observed spectra, we performed full three-dimensional (3D) simulations (details in Methods) and the result is shown in Fig. 2b . The uncertainty in the medium parameters—specifically the material dispersion, Kerr index and ionization rates—over such a large spectrum render quantitative comparison challenging. Nonetheless, we find that the main spectral features are qualitatively reproduced. The simulation confirmed an extended self-channeling behaviour characteristic of filamentation. Supplementary Fig. S1 shows the beam size during propagation in the 2 mm YAG plate for the simulation of Fig. 2b . The beam undergoes several self-focussing events and does not diffract over a distance greater than the Rayleigh range of 1.17 mm. Our observation of massively asymmetric broadening, with the short wavelength edge of the supercontinuum being similar to that observed with visible/near-infrared pumping, is consistent with a simple qualitative picture of supercontinuum generation in bulk materials. In this picture, one mechanism for spectral broadening is self-phase modulation, which produces a spectral shift proportional to the temporal intensity gradient, with red shift on the rising edge and blue on a falling edge. In conjunction with the two main temporal reshaping mechanisms—self-steepening and space-time focussing—a steep trailing edge occurs resulting in a blue shift. Simultaneously, free electrons are produced by ionization throughout the pulse, causing an ultrafast decrease in the refractive index, leading to a blue shift. The effect may be clamped by ionization losses, dispersion, and defocussing. Which of the mechanisms dominate depends strongly on the pulse and material parameters [18] , [19] , [20] . However, these considerations suggest that, as the clamping of the blue shift is largely determined by the material properties, the short wavelength edge of the spectrum may be largely independent of the pump wavelength, explaining the enormous spectra we observe by pumping in the mid-infrared. More rigorous theoretical support for this conjecture comes from a Born approximation-like view of supercontinuum in bulk materials [21] in which the spectral extent is largely determined by the medium dispersion. In this view, the angularly resolved { θ , λ } spectrum is linked to the mechanism through phase-matching. Normal, near-zero or anomalous dispersion manifests in X, fishtail, or O-shaped structures, respectively [22] , [23] , [24] , in the { θ , λ } domain. A comparison between theory and experiment ( Fig. 2a,b ) indeed confirms the phase-matching nature of the process and we overlay results from analytical calculations [22] as black lines in Fig. 2a . The most intense part of the spectrum corresponds to the O-like structure typical of the anomalous dispersion regime. The hyperbolic branch crossing the axis around 560–620 nm corresponds to the fishtail, that is, the loci of phase-matched angle and wavelength lying in the visible region of the spectrum. Simulations show that this tail appears in the last 400 μm of the YAG plate and is not affected by harmonic generation. Switching off harmonic generation in simulations by, for example, propagating the envelope rather than the carrier resolved field only suppresses the peak emerging around 1,100 nm. This also indicates that carrier-envelope phase does not affect the fishtail structure of the spectrum whose features are always present and start with a slightly different focal position with respect to the entrance face of the YAG plate. The fishtail structure also appears with different Kerr coefficients and ionization rates. Increasing n 2 up to a factor of 4 leads to a broader extent of the main spectral peak centred at 3,000 nm and a change in the balance between third-harmonic generation and the supercontinuum. Higher Kerr coefficients lead to a prevailing fishtail with respect to the third harmonic. Although the simulation reproduces the main characteristics of the angularly resolved spectrum, some features are absent such as the third harmonic around 1,100 nm. In fact, the simulations show third-harmonic generation in first millimetre of propagation, but subsequently loses prominence owing to the emergence of the fish tail. 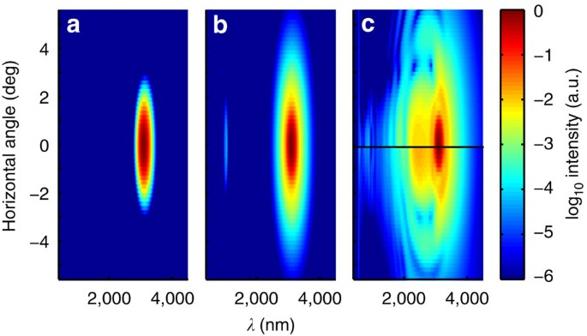Figure 5: Angularly resolved spectra during propagation. Angularly resolved spectra at (a)z=0 mm, (b)z=0.7 mm and (c)z=2 mm, with logarithmic intensity colour scale. In (c), the upper and lower halves show the spectrum without and with averaging over the intensity fluctuations. Figure 5a–c shows angularly resolved spectra at three planes of propagation. In these simulations, the averaging over laser intensity fluctuations used in Fig. 2a has not been performed. By z =0.7 mm, the third-harmonic has formed into an isolated feature, which resembles that observed in the experiment. However, during the subsequent propagation to z =2 mm, the third harmonic undergoes reshaping, driven by the reshaping of the main pulse. This leads to a less distinct feature than observed experimentally. Because the reshaping of the third-harmonic feature involves the interplay of phase matching, the strength of the Kerr index at very different wavelengths, and the reshaping dynamics of the pump, we attribute this discrepancy to small inaccuracies in the simulation parameters that dramatically influence the interplay during filamentation. Figure 5: Angularly resolved spectra during propagation. Angularly resolved spectra at ( a ) z =0 mm, ( b ) z =0.7 mm and ( c ) z =2 mm, with logarithmic intensity colour scale. In ( c ), the upper and lower halves show the spectrum without and with averaging over the intensity fluctuations. Full size image On this basis of the overall agreement between experiment and simulations, we use the latter to examine the output temporal on-axis profile, shown in Fig. 6a . We find that the pulse duration has been reduced by more than a factor of 10 (the satellite peaks are 50% lower in peak intensity), and the main peak has near-single-cycle duration. Pulse compression is known to occur in filamentation [25] but this is the first time that numerics exhibit such a marked compression in a condensed medium. We attribute this mostly to the weak anomalous dispersion at mid-infrared wavelengths, combined with the higher order of the multiphoton ionization processes (with respect to, for example, 800 nm pump pulses) that limit the maximum intensity and enable stronger nonlinear reshaping dynamics. 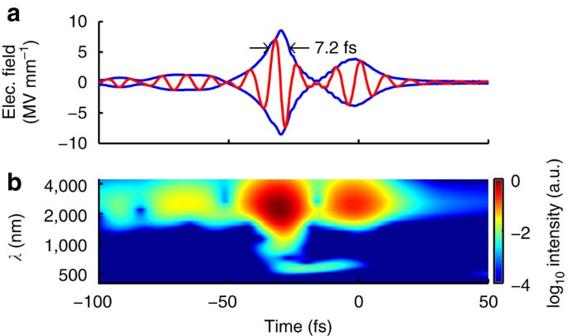Figure 6: Self-compression structure. (a) Temporal profile and spectrogram of output pulse. Temporal envelope (blue) and field oscillations (red) and (b) spectrogram of the on-axis simulated pulse emerging from the YAG plate; note the logarithmic intensity colour and wavelength scale in the spectrogram. Figure 6: Self-compression structure. ( a ) Temporal profile and spectrogram of output pulse. Temporal envelope (blue) and field oscillations (red) and ( b ) spectrogram of the on-axis simulated pulse emerging from the YAG plate; note the logarithmic intensity colour and wavelength scale in the spectrogram. Full size image A more complete picture of the output pulse is given by the spectrogram shown in Fig. 6b . This shows that the short wavelength components, below 1,500 nm, emerge from the output face nearly simultaneously with the main peak. Furthermore the overall time-frequency distribution is simple, containing only a few distinct peaks. Therefore, the numerics indicate the tantalizing possibility of achieving in an extremely simple setting, near-single-cycle and carrier-envelope phase stable pulses using mid-infrared pump lasers. In summary, we demonstrated the first stable multi-octave supercontinuum from filamentation of mid-infrared femtosecond pulses in bulk material. We measured a spectrum spanning 450–4,500 nm, corresponding to 3.3 octaves, with a spectral energy density of 2 pJ nm −1 –10 nJ nm −1 . The smoothness of the spectrum indicates absence of complex pulse splitting and a carrier-envelope phase measurement indicates shot-to-shot reproducibility over a significant spectral range. We obtained an angularly resolved far-field spectrum with the main features captured by full 3D simulations. By demonstrating a simple and robust method for coherently extending the spectrum of an amplified femtosecond mid-infrared pulse to the ultraviolet, we provide a powerful platform for the next generation of ultrafast applications. Stability and f–2f interferometry Figure 3 displays a schematic of the f–2f interferometer used to obtain the data in Fig. 4 . The output of the YAG plate is relay-imaged with a 50-mm focal length CaF 2 lens into a 1-mm thick beta barium borate crystal. Type I phase matching is used to generate the second harmonic of wavelength components around 1,500 nm. The emerging second harmonic as well as fundamental supercontinuum are collimated with another 50-mm focal length CaF 2 lens. After passing a polarizing beamsplitter cube that is oriented at 45° with respect to the polarization axis of the generating mid-infrared beam, the interfering components are recorded with a fibre-coupled silicon CCD spectrometer (Ocean Optics HR4000). The resulting interferogram is shown in Fig. 3 for a 15-s subset recorded over 10 min. Memory limitations dictate an ~1 s break every 4 s during data recording. The interferometric phase is extracted using Fourier filtering [26] . Mathematically, it is given by φ I =2 φ (1,500 nm)− φ (750 nm) where φ ( λ ) is the spectral phase, and is therefore sensitive to both the carrier-envelope phase of the pump laser as well as nonlinear phase shifts introduced during supercontinuum generation. Numerical methods We performed numerical simulations of the nonlinear propagation of the frequency components of the infrared pulse in the YAG plate using a radially symmetric carrier resolving model in the form of the forward Maxwell equation: where z is the propagation coordinate; k ( ω ) and n ( ω ) denote the frequency-dependent wavenumber and refraction index of the medium and account for the chromatic dispersion via a Sellmeier relation [27] . Diffraction is described by the second term on the right hand side of equation (1) in the paraxial approximation, which is well suited to our numerical aperture. The nonlinear polarization is: where the first term describes Kerr self-focussing and third-harmonic generation, and P plasma describes plasma and nonlinear absorption. The plasma contribution is introduced in the model via a current J =− iωP plasma , which is more easily calculated in the temporal domain by resolving the evolution equation for the current density: where ρ denotes the plasma density and τ c the typical electron collision time. Self-steepening and nonlinear chromatic dispersion are accounted for via the frequency dependence of nonlinear source terms in equation (1). The third-order susceptibility is obtained from the nonlinear index coefficient for the optical Kerr effect, n 2 =7×10 −16 cm 2 W −1 (refs 28 , 29 , 30 ). The model is coupled to an evolution equation ∂ t ρ = W ( I )+( σ / U i ) ρE , for the density ρ of the electron-hole and electron-ion plasma [31] generated by optical field ionization and avalanche. Optical field ionization rates W ( I ) for YAG, considered as a condensed medium with ionization potential U i =6.5 eV, follow Keldysh's formulation [32] and are shown in Supplementary Fig. S2 . The avalanche rate follows the Drude model with an estimated collision time of τ c =3 fs, which yields an inverse Bremsstrahlung cross-section σ =2.6×10 −20 cm 2 . Complete analytical formulas are thoroughly presented in ref. 33 . The parameters for the input optical pulse correspond to the experiments. Technical details on the resolution method are exhaustively described in ref. 34 . This carrier resolving model has been applied for the first time to nonlinear propagation and filamentation in YAG in the present work, allowing us to uncover the role of light-bullet and so-called fishtail formation in supercontinuum and conical emissions from a filament pump in the anomalous dispersion region. Comparisons of results with those obtained with more standard envelope propagation models [34] indicated that third-harmonic generation and carrier envelope phase do not have a significant role in the extent of supercontinuum. In particular, the nonlinear envelope equation that does not describe third- and low-order harmonic generation, nevertheless allowed us to capture the generation of a hyperbolic fishtail associated with the green-yellow peak at 550 nm, thus ruling out fifth harmonic generation as a physical process responsible for this peak. We also note that this peak appears in numerical results for a broad range of medium parameters and is tunable in wavelength when medium parameters vary. For example, changing Keldysh's ionization rates into their multiphoton ionization counterparts ( Supplementary Fig. S2 ) leads to a fishtail at 550 nm when the cross-section coefficient is decreased below σ 17 =1×10 −209 s −1 cm 34 W −17 . How to cite this article: Silva, F. et al . Multi-octave supercontinuum generation from mid-infrared filamentation in a bulk crystal. Nat. Commun. 3:807 doi: 10.1038/ncomms1816 (2012).